The bipolar assembly domain of the mitotic motor kinesin-5 An outstanding unresolved question is how does the mitotic spindle utilize microtubules and mitotic motors to coordinate accurate chromosome segregation during mitosis? This process depends upon the mitotic motor, kinesin-5, whose unique bipolar architecture, with pairs of motor domains lying at opposite ends of a central rod, allows it to crosslink microtubules within the mitotic spindle and to coordinate their relative sliding during spindle assembly, maintenance and elongation. The structural basis of kinesin-5’s bipolarity is, however, unknown, as protein asymmetry has so far precluded its crystallization. Here we use electron microscopy of single molecules of kinesin-5 and its subfragments, combined with hydrodynamic analysis plus mass spectrometry, circular dichroism and site-directed spin label electron paramagnetic resonance spectroscopy, to show how a staggered antiparallel coiled-coil ‘BASS’ (bipolar assembly) domain directs the assembly of four kinesin-5 polypeptides into bipolar minifilaments. Accurate chromosome segregation during mitosis is known to underlie the propagation of all life on Earth [1] , [2] . This process depends upon the action of a subcellular bipolar machine, the mitotic spindle, which uses dynamic microtubules (MTs) plus multiple kinesin and dynein motors to generate the piconewton-scale forces required for mitotic movements [2] , [3] , [4] . Of these, the MT-based motor kinesin-5 has a key role, being essential for the assembly of bipolar spindles in most eukaryotic cells and driving or constraining the rate of spindle elongation [5] , [6] , [7] , [8] . Studies of a recombinant vertebrate kinesin-5 motor domain subfragment [6] and a native kinesin-5 holoenzyme purified from Drosophila embryos [9] , [10] , [11] suggest that kinesin-5 is a ‘slow’, plus-end-directed, bipolar, homotetrameric motor capable of using pairs of N-terminal motor domains at opposite ends of a central rod to crosslink MTs into bundles. Moreover, sophisticated motility assays reveal that single vertebrate [12] and Drosophila [13] kinesin-5 holoenzymes can crosslink and slide adjacent MTs, displaying a three-fold preference for MTs in the antiparallel versus the parallel orientation. Together, these data support the hypothesis that kinesin-5 functions via a ‘sliding filament’ mechanism, cross-linking adjacent MTs into bundles throughout the spindle, and exerting outward forces on antiparallel MTs to drive bipolar spindle assembly, poleward flux and anaphase B spindle elongation [14] , [15] , [16] . In this model, the assembly of four kinesin-5 polypeptides into a bipolar minifilament is crucial, but the molecular basis of this arrangement, which is unique among MT-based motor proteins, remains unclear. This could be clarified by the determination of an improved, ideally atomic resolution understanding of kinesin-5’s structure, but in practice this proves to be difficult. So far, for example, we have failed to crystallize kinesin-5 for structure determination by X-ray diffraction, probably because of the molecule’s asymmetry. Therefore, we have adopted an alternative approach involving a combination of electron microscopy, hydrodynamic analysis and various spectroscopy procedures to obtain structural data on the BASS domain of this key mitotic motor. 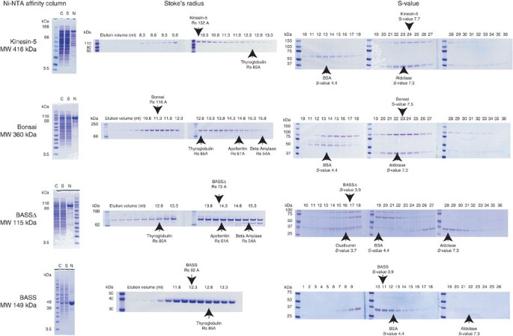Figure 1: Purification steps and hydrodynamic analysis. The left panels show SDS–PAGE analysis of samples from different steps of purification of each protein. Samples are crude extract (C), supernatant after application to Ni-NTA column (S) and Ni-NTA column eluate (N). Molecular weight values of some of the MW markers are given next to the corresponding band for comparison. Middle panels include the SDS–PAGE analysis of fractions from gel filtration column Superose6 10/300 GL (each fraction is 0.25 ml eluted at a flow rate of 0.25 ml min−1). The Stoke’s radius (Rs) of some of the standard proteins and the calculatedRsof the samples are indicated by arrows. The right panels contain SDS–PAGE analysis of fractions from sucrose density gradients. Each fraction is 0.25 ml from a 12 ml 5–20% linear sucrose gradient. The sedimentation coefficients (S-value) of some of the standard proteins and the calculatedS-values of each sample are indicated by arrows. The BASS domain directs bipolar homotetramer assembly We examined the oligomeric state, ultrastructure and dimensions of baculovirus-expressed and purified Drosophila kinesin-5 (aka KLP61F) and several truncated mutants thereof using hydrodynamic analysis combined with electron microscopy ( Figs 1 , 2 , 3 ; Table 1 ; Supplementary Fig. S1 ). We found that transmission electron microscope (TEM) and scanning TEM (STEM) of proteins that were negatively stained with uranyl formate (UF) immediately following gel filtration ( Fig. 1 ) yielded high-quality images ( Fig. 2 ). As each preparation contained a poly-histidine tag on either the N- or C-terminal end, the relative orientation of individual kinesin-5 subunits within these preparations could be determined by decoration with 2 and 5 nm Ni-NTA-nanogold particles before EM ( Fig. 3 ). Figure 1: Purification steps and hydrodynamic analysis. The left panels show SDS–PAGE analysis of samples from different steps of purification of each protein. Samples are crude extract (C), supernatant after application to Ni-NTA column (S) and Ni-NTA column eluate (N). Molecular weight values of some of the MW markers are given next to the corresponding band for comparison. Middle panels include the SDS–PAGE analysis of fractions from gel filtration column Superose6 10/300 GL (each fraction is 0.25 ml eluted at a flow rate of 0.25 ml min −1 ). The Stoke’s radius ( R s ) of some of the standard proteins and the calculated R s of the samples are indicated by arrows. The right panels contain SDS–PAGE analysis of fractions from sucrose density gradients. Each fraction is 0.25 ml from a 12 ml 5–20% linear sucrose gradient. The sedimentation coefficients ( S -value) of some of the standard proteins and the calculated S -values of each sample are indicated by arrows. 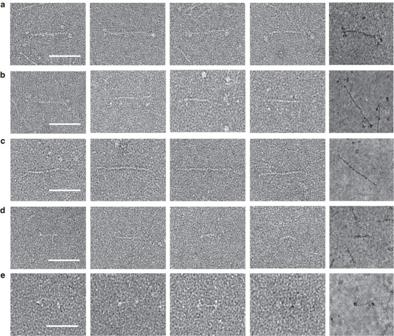Figure 2: EM images of the undecorated constructs. (a) N-terminally His-Tagged Kinesin-5 (N-FL), (b) C-terminally His-tagged Kinesin-5 (C-FL), (c) ML-Kinesin-5, (d) BASS domain (BASS) and (e) Bonsai construct. The horizontal panels 1–4 are TEM images followed by a panel of STEM images of the same sample. The scale bar corresponds to 50 nm. (SeeSupplementary Figs S2 and S5for representative undecorated images—due to space constraints only N-FL and Bonsai are shown). Full size image Figure 2: EM images of the undecorated constructs. ( a ) N-terminally His-Tagged Kinesin-5 (N-FL), ( b ) C-terminally His-tagged Kinesin-5 (C-FL), ( c ) ML-Kinesin-5, ( d ) BASS domain (BASS) and ( e ) Bonsai construct. The horizontal panels 1–4 are TEM images followed by a panel of STEM images of the same sample. The scale bar corresponds to 50 nm. (See Supplementary Figs S2 and S5 for representative undecorated images—due to space constraints only N-FL and Bonsai are shown). 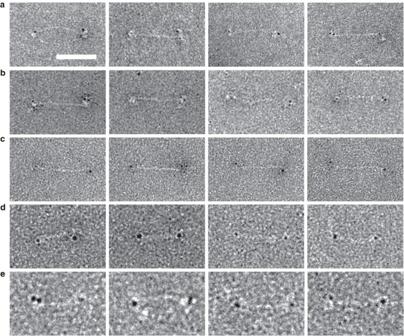Figure 3: TEM images of 2 nm Nanogold decorated constructs. (a) N-terminally His-tagged kinesin-5 (N-FL), (b) C-terminally His-tagged kinesin-5 (C-FL), (c) ML-kinesin-5, (d) BASS domain (BASS) and (e) Bonsai construct. The 2 nm Nanogold particles are seen as black dots at the HisTag positions. The scale bar corresponds to 50 nm fora,b,c; 25 nm ford,e. (seeSupplementary Figs S3, S4, S6for representative decorated images—due to space constraints, not all constructs are shown). Full size image Figure 3: TEM images of 2 nm Nanogold decorated constructs. ( a ) N-terminally His-tagged kinesin-5 (N-FL), ( b ) C-terminally His-tagged kinesin-5 (C-FL), ( c ) ML-kinesin-5, ( d ) BASS domain (BASS) and ( e ) Bonsai construct. The 2 nm Nanogold particles are seen as black dots at the HisTag positions. The scale bar corresponds to 50 nm for a , b , c ; 25 nm for d , e . (see Supplementary Figs S3, S4, S6 for representative decorated images—due to space constraints, not all constructs are shown). Full size image Table 1 Hydrodynamic analysis results and native molecular weight of full-length Kinesin-5, Bonsai, BASSΔ and BASS constructs. Full size table Full-length (FL) and motorless (ML) kinesin-5 constructs are homotetrameric MT-cross-linking proteins [13] , [17] . In the EM, undecorated FL-kinesin-5 molecules were observed to be 79 nm long dumbbell-shaped molecules, containing a central 57 nm long × 3.1 nm diameter rod, from which two distinct 8.1 × 5.5 nm globular domains emerged ( Fig. 2 , Supplementary Figs S1–S3 ). In favourable STEM images (for example, Fig. 2a , right hand panels) fine linkers appeared to attach the globular domains to the rod. Molecules tagged with poly-histidine on either the N-terminal motor domain or on the C-terminal tail were efficiently decorated on both ends with nanogold particles ( Fig. 3 , Supplementary Figs S1b and S3 ). ML-kinesin-5 consisted of bipolar filaments of the same diameter as the rod of FL-kinesin-5, but significantly longer (73.4 nm) and lacking globular domains at both ends ( Figs 2 and 3 ; Supplementary Figs S1 and S4 ). These results confirm that kinesin-5 is bipolar with pairs of motor domains linked to a central rod. Moreover, the observation that ML-kinesin-5 is longer than the rod of FL-kinesin-5 suggests that, in the intact holoenzyme, the C-terminal tail domains may fold up to interact with the N-terminal motor domains, and this may have functional consequences (see Discussion ). In preliminary studies, we identified a region comprising residues 631–920 of the kinesin-5 rod as the shortest subfragment capable of assembling into homotetramers [17] ( Supplementary Fig. S1a ). This subfragment, which for reasons described below we now refer to as the BASS domain, was highly purified ( Fig. 1 ) and examined by EM where it was observed to comprise 32 nm long rods whose four subunits are arranged in an antiparallel fashion based on nanogold decoration ( Figs 2 and 3 , Supplementary Figs S1 and S6 ). To evaluate the role of this BASS domain in the assembly of four FL-kinesin-5 subunits into bipolar homotetramers, we engineered and purified two new deletion constructs, a ‘Bonsai’ construct (analogous to the Bonsai subfragment of the kinetochore protein, NDC80 (ref. 18 )), which contains the BASS domain and motor domains but lacks the N-terminal half of the rod, and a BASS-Δ subfragment, which lacks the BASS domain but contains the entire remainder of the kinesin-5 polypeptide chain ( Fig. 1 ; Supplementary Fig. S1 ). Remarkably, the Bonsai construct appeared to assemble into short, dumbbell-shaped bipolar homotetramers, 38 nm in length (although at low concentration, <1 mg ml −1 , a small amount of dimeric Bonsai was also detected by gel filtration but was not studied further), whereas the BASS-Δ subfragment only formed monomers ( Figs 1 , 2 , 3 ; Table 1 ; Supplementary Figs S1 and S5 ). Thus, we feel justified in referring to residues 631–920 as the BASS (for bipolar assembly) domain, because it is essential for bipolar homotetramer assembly— kinesin-5 and all subfragments that contain it assemble into bipolar homotetramers, whereas subfragments that lack it form monomers. Fitting the BASS domain into the kinesin-5 rod We initially hoped to use X-ray diffraction to directly determine the molecular mechanism by which the BASS domain specifies the unique bipolar architecture of kinesin-5, but in extensive robotic trials this elongated asymmetric molecule did not crystallize. Thus, instead, we tried to develop a simple model for how the 32 nm long BASS domain is arranged within a 57-nm long kinesin-5 rod domain. The sequence of each 1,066 residue Drosophila kinesin-5 subunit predicts that it consists of globular motor and unstructured tail domains, separated by a 566 residue rod (residues 354–920) [17] , [19] ( Supplementary Fig. S1 ). The rod domain is predicted to be 95–97% α-helical, including several coiled-coil (CC) segments interrupted by only 3–5% random coil breaks (using paircoil2 programme; Supplementary Fig. S8a ). Thus, the above TEM data are consistent with four kinesin-5 subunits forming some kind of four-strand helical bundle. This line of reasoning led us to favour an antiparallel arrangement of two parallel CCs for the BASS domain, in which the N-terminal ends overlap to form an antiparallel 4-strand core, leaving single C-terminal CC overhangs at either end (Fig. 6) as in a vimentin tetramer [20] . Assuming 0.15 nm per residue, if residue 630 of one CC lies in register with residue 809 of its antiparallel neighbour, this arrangement would produce a structure that is predicted to be ≈60 nm long like the kinesin-5 rod. Such a BASS domain would fit the dimensions of the rod of FL-kinesin-5, but it is inconsistent with the smaller lengths of the 32 nm long BASS domain observed by EM ( Figs 2 and 3 and Supplementary Fig. S1 ). Actually, based on length considerations alone, a parallel arrangement of four polypeptide chains with residues from 354 to 920 lying in register all along the rod domain superficially gives a better fit to the data. This predicts an 85-nm rod for FL-kinesin-5, which is 49% longer that the 57 nm rod observed ( Supplementary Fig. S1 ). This is reasonable given that similar arguments for kinesin-1 predict a rod that is 28% longer than that observed [21] , [22] , [23] . The BASS domain and Bonsai would have residues 354–630 deleted from the N-terminal ends of all four chains, producing a 43-nm long rod, which is more consistent with lengths of the 32 nm BASS domain and 38 nm Bonsai, but of course such a parallel arrangement cannot be reconciled with our current nanogold and previous IgG decoration. But adding to the puzzle, the 3 nm diameter of the negatively stained kinesin-5 rod observed by EM ( Supplementary Fig. S1 ) lies within the range expected of a four helix bundle yet, according to at least one report, this is also the diameter of the negatively-stained class II myosin rod, which is a single parallel CC assembled from two, rather than four polypeptide chains [24] . These considerations made us wonder if some systematic experimental error in our analysis of kinesin-5’s architecture was misleading us, prompting us to further test and refine our antiparallel CC model for the kinesin-5 BASS domain. Consolidating the homotetrameric state of the BASS domain Our estimate of four subunits per kinesin-5 (refs 9 , 17 ) ( Fig. 1 , Table 1 ) could be compromised by the high Stokes radius of FL-kinesin-5, which causes it to elute from gel filtration columns in a position that is hard to calibrate. This is less of a concern for the smaller BASS domain, which by analytical ultracentrifugation (AUC) [25] displayed an S -value of between 3.5 and 4S (extrapolated to zero concentration), in very good agreement with the value of 3.9S estimated using routine sucrose density gradient centrifugation ( Supplementary Fig. S7 ). However, even this relatively small subfragment can display non-ideal behaviour when migrating in a centrifugal field due to: (i) its high charge and (ii) its high frictional ratio ( f / f 0 =2.6) reflecting an asymmetric, elongated shape, consistent with EM ( Figs 2 and 3 ). Both these effects give rise to a hyper-sharpening of the sedimenting protein boundary, which impedes accurate determination of the diffusion coefficient for direct MW determination by AUC. Mass spectrometry was used to further test the oligomeric state of the BASS domain ( Fig. 4a ). Under denaturing conditions, a single kinesin-5 subunit displayed MW=34,535.5 Da. Mass spectra obtained under non denaturing conditions yielded ions with masses virtually identical to the theoretical values for the monomer (34,534.9 Da versus 34,629.9 Da; 0.28% error) as well as for corresponding dimers (69,069.9 Da versus 69,356.3 Da; 0.41% error); and tetramers (138,139.8 Da versus 138,974 Da; 0.6% error). We also detected a BASS-dimer that was contaminated with the chaperone HSP70, albeit at a very low level assuming equal ionization efficiency. Also, as the small species’ were not detected in routine hydrodynamic analyses ( Fig. 1 ; Table 1 ), it seems reasonable to propose that the BASS domain is a tetramer that dissociates into dimer and monomer under the conditions used for MS. 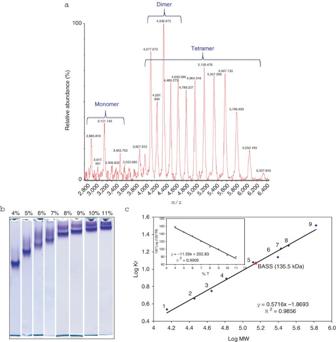Figure 4: Molecular weight determination of the BASS domain by mass spectrometry and native PAGE. (a) Mass spectrum of the BASS domain measured on SYNAPT G2 HDMS under native-like conditions (b) Native PAGE was performed at eight different acrylamide concentrations for purified BASS (5 μg protein loaded into each lane) along with all the standards. Each lane represents a lane from a gel of different %T as indicated. The lanes were cut out from the original photos and aligned for comparison. (c) Standard curve drawn for an individual experiment. The relationship between the retardation coefficient (Kr) values determined for each standard protein and corresponding molecular weights were plotted in a logarithmic scale as a standard curve (R2=0.9856). The MW of BASS is marked with a red square on the standard curve. According to the result of three independent native PAGE experiments the MW of BASS is 153±16 kD. The inset shows a Ferguson plot for the BASS domain (semi logarithmic graph 100 × log(100 ×Rf) versus %T).Rfand LogRfvalues were multiplied by a factor of 100 to avoid negative values in the graphs. Graph shows the relationship between relative mobility of BASS and acrylamide concentration (R2=0.9905). The slope of the line representsKrfor BASS domain. The molecular weight standards as numbered in the Figure are given in the methods section. Figure 4: Molecular weight determination of the BASS domain by mass spectrometry and native PAGE. ( a ) Mass spectrum of the BASS domain measured on SYNAPT G2 HDMS under native-like conditions ( b ) Native PAGE was performed at eight different acrylamide concentrations for purified BASS (5 μg protein loaded into each lane) along with all the standards. Each lane represents a lane from a gel of different %T as indicated. The lanes were cut out from the original photos and aligned for comparison. ( c ) Standard curve drawn for an individual experiment. The relationship between the retardation coefficient ( K r ) values determined for each standard protein and corresponding molecular weights were plotted in a logarithmic scale as a standard curve ( R 2 =0.9856). The MW of BASS is marked with a red square on the standard curve. According to the result of three independent native PAGE experiments the MW of BASS is 153±16 kD. The inset shows a Ferguson plot for the BASS domain (semi logarithmic graph 100 × log(100 × R f ) versus %T). R f and Log R f values were multiplied by a factor of 100 to avoid negative values in the graphs. Graph shows the relationship between relative mobility of BASS and acrylamide concentration ( R 2 =0.9905). The slope of the line represents K r for BASS domain. The molecular weight standards as numbered in the Figure are given in the methods section. Full size image We also used a 3rd method, native PAGE, in which the BASS domain migrates under the influence of an electric, rather than a centrifugal, field ( Fig. 4b ). We estimated the BASS domain’s molecular weight using Ferguson plots [26] to be 153±16 kD based on three independent sets of experiments, again highly consistent with it being a tetramer and supporting the results of hydrodynamic analyses ( Table 1 ). No dimeric or monomeric species’ were detected, although a very small amount of aggregated protein (<10% by mass) was detected at high crosslinker percentages. Thus, we feel confident that the BASS domain of kinesin-5 is a homotetramer. EPR spectroscopy of the BASS domain The possibility that some of the predicted CC segments within the kinesin-5 rod domain, described above, do not reflect the true structure of this region of the molecule is underscored by our observation that the BASS-Δ subfragment is monomeric. This raises the possibility that the predicted CCs seen in regions of the rod lying outside the BASS domain [17] , are in fact single alpha helical or disordered domains like those seen in some myosins [27] . Therefore, based on elegant studies of vimentin [28] , we decided to use site-directed spin labelling and electron paramagnetic resonance (SDSL-EPR) spectroscopy and homology modelling to test the CC predictions and to investigate sites of interaction between side chains of adjacent CCs within the BASS domain. For SDSL-EPR, we created 118 spin-labelled mutants spanning four regions, that is, region 1=aa 642–671; 2=700–719; 3=776–835; 4=852–859 ( Supplementary Fig. S8a,b ) that represent 40% of the BASS domain. This was done using a mutant BASS domain, BASS-NoC, in which all Cys residues were changed by site-directed mutagenesis to Ser, as a template for creating these single Cys mutants. All 118 mutants were spin-labelled with S-(2,2,5,5-tetramethyl-2,5-dihydro-1H-pyrrol-3-yl)methyl methane sulfonothioate, (MTSL) and examined by EPR. Our aim was to verify residues in the ‘a’ and ‘d’ positions of the CC heptad repeat (a–g) as these positions appear uniquely in a series within two parallel strands of a single CC. Thus, spin labels placed on ‘a’ and ‘d’ side chains are closely packed in the hydrophobic core of the CC and are thereby strongly immobilized and magnetically coupled, giving rise to a shallow EPR spectrum characterized by broad peaks. As a control, SDS-induced denaturation disrupts these interactions, producing a sharper spectrum (tight peaks) indicating a mobile spin label. Two examples are shown in Fig. 5 , which identifies residues 657–671 in region 1 ( Fig. 5a ) and 776–788 in region 3 ( Fig. 5b ) as likely CCs, where the spin-labelled hydrophobic residues in the ‘a’ and ‘d’ positions yielded the expected ‘shallow’ EPR spectrum. In contrast to aas 776–788, residues 796–835 in region 3 did not yield evidence of a CC. Overall aas 657–671 appear more rigid than aas 776–788. EPR spectra for aas 708–719 in region 2 also verified interactions between residues in the a and d positions, but region 4 appears disordered throughout. 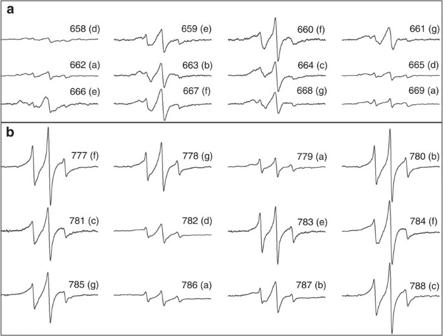Figure 5: EPR spectrum of selected BASS cysteine mutants. The spectrum of selected single cysteine mutants in the first (a) and third (b) CC region are shown. The numbers given on the upper right indicate the location of the cysteine in BASS sequence. The letters (a–g) given in the parenthesis correspond to the position of these residues in the heptad repeat pattern. Note the band broadening at each ‘a’ and ‘d’ positions in the heptad repeat pattern. Comparison of first and third CC region shows that the first region is tighter reflected by the amplititude of spectra. At positions where the spin can move freely the EPR spectra have a higher amplititude. Figure 5: EPR spectrum of selected BASS cysteine mutants. The spectrum of selected single cysteine mutants in the first ( a ) and third ( b ) CC region are shown. The numbers given on the upper right indicate the location of the cysteine in BASS sequence. The letters (a–g) given in the parenthesis correspond to the position of these residues in the heptad repeat pattern. Note the band broadening at each ‘a’ and ‘d’ positions in the heptad repeat pattern. Comparison of first and third CC region shows that the first region is tighter reflected by the amplititude of spectra. At positions where the spin can move freely the EPR spectra have a higher amplititude. Full size image These data were used to refine the antiparallel CC model for the BASS domain. In a search using Rosetta software, the protein structure displaying the greatest homology with the BASS domain was the classic CC protein, tropomyosin [29] (20% match). The CC structure predicted from this ‘hit’ was refined according to the constraints of the CCs determined by the EPR data and assembled into a staggered antiparallel CC based on the aforementioned biochemical and EM data. The resulting antiparallel tetramer model was further tested using two sets of single and double mutants that form tetramers based on hydrodynamic analysis (Fig. 7). The first of these contain Cys at residues 671 (position g) and 791 (position b), which are predicted to be juxtaposed within neighbouring antiparallel CCs in the model. Single mutants in which either one of these Cys residues is spin-labelled with MTSL display sharp peaks in EPR spectra (Fig. 7a inset). However, in double mutants, when both these positions are spin-labelled, their EPR spectra reveal evidence of strong interactions (spins are <1.5 nm apart), giving rise to peak broadening in the spectrum (compare black and red lines in Fig. 7a; left spectra). If the BASS domain consisted of a pair of parallel, in register CCs derived from the kinesin-5 rod mentioned above, these residues would be 18 nm apart and their spin labels could not interact in this way. Identical experiments performed with mutants containing Cys residues at positions 671 and 788 (only three residues upstream of 791) provided no evidence of interaction (data not shown). This analysis yielded a model for the BASS domain in which the tetrameric antiparallel overlap zone has N-terminal residue 630 of one CC lying in register with residue 835 of its antiparallel partner, leaving residues 835–920 to form 85 residue single parallel CC overhangs at both ends ( Fig. 6a ). It is striking that the three CCs verified by SDSL-EPR spectroscopy all lie within the central overlap zone, yet aas 852–859 lying within the overhangs, which displays a high probability of CC formation based on sequence analysis, is unlikely to form a CC based on the EPR analysis ( Fig. 6b ). Moreover, CD spectroscopy of the BASS domain yields a classic α-helical spectrum with minima at wavelengths of 208 and 222 nm ( Supplementary Fig. S8c ), but when these data were quantified [30] we estimated that the BASS domain was only 50% α-helical (on average 48.8±1.5% α helix, 6.7±1.6% β-sheet, 14.0±1.9% turn and 30.5±1.2% random coil). Based on these data we propose that within the purified BASS domain protein, the overhangs become disordered, reducing the overall CC and single alpha helical content of the protein, and rendering the overhangs invisible by electron microscopy. This is consistent with the superposition of the BASS domain model onto STEM images, where only the central overlap zone is visible ( Fig. 6c , right hand panels). 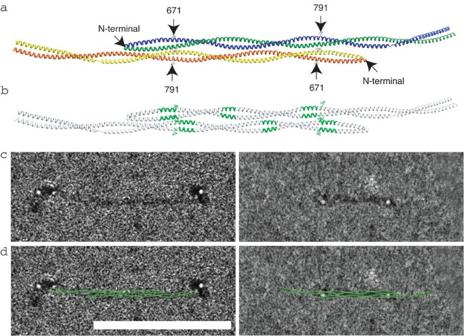Figure 6: Homology Model for BASS and superimposition onto the EM data. (a) Homology model of BASS. Black arrows point to the N-terminal end of the parallel dimers. Rosetta modelling was used to construct the model and EPR data were used to refine it. The spins are shown on residue 671 and 791 (indicated by arrows) for the orientation of the chains. According to the model parallel dimers form a tetramer in an antiparallel fashion. The dimer region extending out from tetrameric core starts around residue 835. Each strand of BASS domain is shown with a different colour (b). The homology model; all strands are shown in white and the CC regions supported by EPR analysis are highlighted in green. The regions are between residues 657–671, 708–719 and 776–788. (c) STEM image of full-length Kinesin-5 (left) and BASS (right) decorated with 2 nm Nanogold particles. (d) Superimposition of the homology model on the stem images shown in (c) by taking into account the dimensions of the model. The 2 nm Nanogold decoration at the N-terminus of the BASS matches with the N-terminal location in the homology model. Figure 6: Homology Model for BASS and superimposition onto the EM data. ( a ) Homology model of BASS. Black arrows point to the N-terminal end of the parallel dimers. Rosetta modelling was used to construct the model and EPR data were used to refine it. The spins are shown on residue 671 and 791 (indicated by arrows) for the orientation of the chains. According to the model parallel dimers form a tetramer in an antiparallel fashion. The dimer region extending out from tetrameric core starts around residue 835. Each strand of BASS domain is shown with a different colour ( b ). The homology model; all strands are shown in white and the CC regions supported by EPR analysis are highlighted in green. The regions are between residues 657–671, 708–719 and 776–788. ( c ) STEM image of full-length Kinesin-5 (left) and BASS (right) decorated with 2 nm Nanogold particles. ( d ) Superimposition of the homology model on the stem images shown in ( c ) by taking into account the dimensions of the model. The 2 nm Nanogold decoration at the N-terminus of the BASS matches with the N-terminal location in the homology model. Full size image We reasoned that deletion of the 85 aa C-terminal overhangs might yield a smaller tetrameric ‘core’ and this was tested biochemically by expression and purification of BASS-core (BASS 631–835), which does indeed behave as a stable homotetramer in hydrodynamic analysis, yielding a monodisperse peak in gel filtration in support of the model ( Fig. 7b , Table 1 ; although under conditions used for EM, this fragment tended to aggregate so it has not been further analysed). In contrast, deletion of 120 residues from the C-terminus yielded an unstable core (BASS 631–790) that formed both tetramers and dimers under the same conditions ( Fig. 7b ). 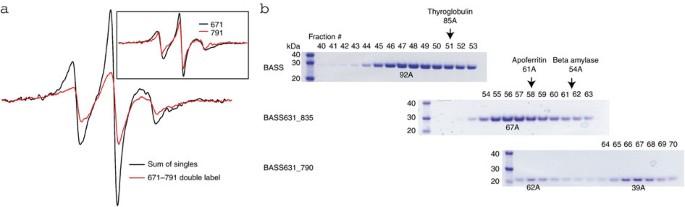Figure 7: Testing the homology model. (a) EPR of double mutants. The panel shows the interaction of the spins at positions 671 and 791. The spectrum from the double mutant has a lower amplitude than the sum of the single mutants (shown in inset). If there was no interaction between the labels at positions 671 and 791, the spectrum from double labelled BASS would resemble the sum of spectra from single labelled protein. (b) Hydrodynamic analysis of truncated BASS proteins. Elution profiles of BASS, BASS631_835 and BASS631_790 from the gel filtration column (Superose6 GL10/30). Fraction numbers are given above each lane. The elution profiles are aligned for ease of comparison between the samples and the Stoke’s radii of the standard proteins are shown. Stoke’s radii of the BASS samples are given below each peak. BASS and BASS631_835 are eluted as monodisperse tetrameric peaks. BASS631_790 eluted in two peaks corresponding to dimer and tetramer species, of which the dimer species is the dominant species based on band intensity and the tetramer form is unstable. Figure 7: Testing the homology model. ( a ) EPR of double mutants. The panel shows the interaction of the spins at positions 671 and 791. The spectrum from the double mutant has a lower amplitude than the sum of the single mutants (shown in inset). If there was no interaction between the labels at positions 671 and 791, the spectrum from double labelled BASS would resemble the sum of spectra from single labelled protein. ( b ) Hydrodynamic analysis of truncated BASS proteins. Elution profiles of BASS, BASS631_835 and BASS631_790 from the gel filtration column (Superose6 GL10/30). Fraction numbers are given above each lane. The elution profiles are aligned for ease of comparison between the samples and the Stoke’s radii of the standard proteins are shown. Stoke’s radii of the BASS samples are given below each peak. BASS and BASS631_835 are eluted as monodisperse tetrameric peaks. BASS631_790 eluted in two peaks corresponding to dimer and tetramer species, of which the dimer species is the dominant species based on band intensity and the tetramer form is unstable. Full size image In the almost two decades since the bipolar, homotetrameric structure was proposed for the mitotic motor, kinesin-5 (refs 9 , 10 ), progress has been made in the structural analysis of its motor domain [31] , [32] but very little has been learned about how it adopts its unique architecture. Thus, the most significant advance of the current study is in providing an advance in that direction, by suggesting how the BASS domain of kinesin-5 can specify how its four subunits assemble into this bipolar organization, which is thought to underlie the sliding filament mechanism by which kinesin-5 functions during mitosis. The idea that the BASS domain forms a four-strand bundle consisting of two antiparallel CC, superficially resembling a vimentin tetramer, is supported by sequence analysis, EM, mass spectrometry, hydrodynamics, native PAGE and site-directed spin label EPR spectroscopy. The results are all incorporated into the summary showing the homology model ( Fig. 6a ) superimposed on STEM images of single molecules of FL-kinesin-5 (left) and the BASS domain (right), decorated on their N-termini with 2 nm Nanogold ( Fig. 6c ). The BASS domain forms a structure that fits very well into the four-strand antiparallel α-helical CC rod of the FL-kinesin-5 homotetramer, but in the EM, the α-helical C-terminal overhangs are apparently not resolved (discussed below). A rigorous test of this model versus alternative 4-strand helical bundle motifs would benefit from an atomic structure. For this it is conceivable that the tetrameric BASS-core, identified herein via predictions based on the BASS domain model, might be a useful target for crystallization. However, the BASS-core displays evidence of instability and under conditions used for EM it tended to form aggregates. Thus, we feel more work must be done to better stabilize this protein in its tetrameric state, before undertaking such detailed structural studies. Previously, we reported that native kinesin-5 purified from Drosphila embryos and examined by rotary shadow EM displayed overall length=96 nm (versus 79 nm herein) with a 61 nm rod (versus 57 nm herein). Moreover, in that study the motor and tail domains appeared collapsed into a single 22 nm globular domain and bipolarity was inferred based on 46 of 70 molecules being decorated on both ends by motor domain-specific IgG [10] . In the current study, the higher yield of purified baculovirus-expressed motor combined with the use of superior UF-negative staining allowed >10-fold more decorated and undecorated molecules, manipulated in various ways, to be examined (for example, for FL-kinesin-5; 530 of 663 molecules were decorated on both ends) and the motor domains could be clearly resolved in favourable images ( Fig. 2 ; Supplementary Fig. S1 ). The revised dimensions and constructs reported here may prove useful for advancing our understanding of kinesin-5 structure and function in the spindle by EM. For example, experiments are in progress to test the prediction that functionally replacing the native KLP61F gene with the gene expressing the Bonsai construct will decrease the length of putative kinesin-5 crossbridges between MTs in embryo mitotic spindles from 60 to 30 nm (ref. 33 ). One unresolved question is why the C-terminal overhangs are not visible in EM images of the BASS domain, where one might expect them to project as single CC rods from the tetrameric BASS-core, and of the Bonsai construct, where they might extend beyond the motor domains on the N-terminal end of the antiparallel neighbouring CCs ( Fig. 6 ). The EM techniques we use should resolve single CCs, so we suspect that, following BASS domain purification, in the absence of their antiparallel neighbour, these overhangs become unstable, disordered and splay apart, making them difficult to visualize by TEM. This speculation is supported by analysis of the purified BASS domain by CD spectroscopy, which yields only 50% α-helix and by SDSL-EPR spectroscopy which fails to detect the predicted CC segments in the overhangs. It is possible that the CD spectrum could underestimate the true α-helical content of the purified BASS domain, much like the kinesin-1 rod, which is estimated to be 65–70% α-helical by CD spectroscopy at physiological temperatures, but is predicted to be 90% α-helix based on sequence analysis [23] . However, this would not be inconsistent with our proposal that the rod of full-length kinesin-5 is largely an alpha helical, antiparallel CC rod, whose CC conformation is preserved in the overlap zone of the BASS domain following its purification ( Fig. 6 ), but not in the overhangs, which become disordered, accounting for the CD, EPR and EM data. In the case of Bonsai, the overhangs also contain the C-terminal tail domain, which we suspect interact with the antiparallel CC’s N-terminal heads, further obscuring their visualization. Indeed, interactions between the C-terminal tails on one CC with the N-terminal heads on the neighbouring CC at each end of the FL-kinesin-5 could explain the curious observation that the tail domains of kinesin-5 are required for MT–MT-cross-linking and sliding by kinesin-5 (ref. 34 ). As the tail domains appear to have MT-binding activity [35] , one explanation for this result is that the kinesin-5 subunits are arranged in parallel and crosslink and slide MTs using a similar geometry to kinesin-1 and kinesin-14 (refs 36 , 37 ), but a head-tail interaction within the kinesin-5 homotetramer suggests that the tails could mediate an allosteric activation of MT binding by the heads instead [34] . As a precedent, head-tail interactions are well established in the case of the better characterized kinesin-1 (ref. 38 ). By EM, the ML-kinesin-5 tetramer is much longer than the rod of FL-kinesin-5, again consistent with the idea that the tail may fold up as a result of its interactions with the motor domain, and the idea that this may have a stabilizing effect is supported by our inability to purify and characterize the ‘tailless’ kinesin-5 complex (this report) [13] . Although this study provides strong support for the bipolar, homotetrameric architecture of kinesin-5 by providing a structural explanation for the organization of the BASS domain, it is important to notice that we also detected other oligomeric states of kinesin-5 and its subfragments in some experiments. For example, the BASS-Δ subfragment only formed monomers, whereas monomer, dimer and tetramer forms of the BASS domain were detected by MS, and in routine hydrodynamic analyses we found some BASS domain dimers co-existing with tetramers. By EM a significant fraction (20% or less) of mono- or un-decorated molecules are seen. Also, in native PAGE and AUC, 2–3% higher order aggregates were detected. Although it is plausible that these are experimental artifacts, it is also possible that they represent functionally distinct oligomeric states that merit further investigation. For example, the formation of higher order filaments analogous to muscle thick filaments might be relevant to the proposal that kinesin-5 acts in concert with a ‘spindle matrix’ [6] , [39] and dimeric or monomeric kinesin-5 could mediate chromosome congression, [40] or contribute to protein synthesis on the ribosome [41] processes for which the functional advantage of a bipolar homotetrameric architecture is not obvious. In summary, this paper reports a major advance in our understanding of how kinesin-5 acquires its unique bipolar architecture. Thus, it represents a significant advance towards the ultimate goal of an atomic resolution understanding of the kinesin-5-dependent sliding filament mechanism that is proposed to underlie key aspects of mitosis and chromosome segregation, processes that are crucial to the formation and maintenance of all known living organisms. Purification of proteins In order to facilitate the purification of the proteins expressed from cloned genes (see Supplementary Methods ) they were 6 × His-tagged either on C- or N-terminal ends. The expression of proteins was done in baculovirus system using SF9 cells as host cells [17] . After 2 days of infection with the corresponding bacmid the cells are harvested by centrifugation. The cell pellet is either used immediately for purification or kept at −80 °C until use. The cell pellet from a 400-ml cell culture is resuspended in 40 ml of Lysis buffer (10 mM Tris–HCl pH 8.0 containing 300 mM KCl, 20 mM Imidazole, 0.2 mM MgCl2, 1 mM PMSF, 1 μg ml −1 pepstatin, 1 μg ml −1 leupeptin, 2 μg ml −1 aprotinin, 20 μg ml −1 benzamidine and 40 μg ml −1 Nα-p-Tosyl- L -arginine methyl ester hydrochloride (TAME)). The lysate was then centrifuged at 37,000 r.p.m. in a Beckman Ultracentrifuge in JS 40.2Ti type rotor. The supernatant was applied to Ni-NTA beads (1.5 ml beads for each batch of SF9 cells from 400 ml culture). The samples from Ni-NTA affinity chromatography were applied to Superose6 GL10/30 gel filtration column. The fractions containing the proteins were analysed by SDS–PAGE and Coomassie Blue staining. EM sample preparation Fresh protein directly from gel filtration was diluted to 2.5 μg ml −1 for full-length and ML constructs or 5 μg ml −1 for the BASS domain with Buffer L. Two microliter of diluted protein was added to a glow discharged holey carbon double film (Cu-400HD, Pacific Grid-Tech), allowed to adsorb for 10 s, washed two times with 40 μl drops of Buffer L with no ATP, then two times with 40 μl drops of water and finally stained with two 40 μl drops of freshly made 0.75% UF [42] before air drying. For gold decorated protein, 1.8 and 5 nm Ni-NTA-Nanogold (Nanoprobes, Inc.) was added to the protein in a molar ratio of 3:1 (ref. 43 ). In order to reduce aggregation caused by the gold cross-linking multiple motors, the gold was added to dilute protein and immediately mixed with three 0.5 s vortex pulses. The reaction was then placed on ice for 15 min and subsequently applied to EM grids as described above. Electron microscopy TEM images were taken on a JEM-2100F TEM (JEOL, Japan) operated at 200 KeV. Micrographs were recorded at a nominal magnification of X50,000 with a 4,096 × 4,096 pixel CCD camera (TVIPS, Gauting, Germany) at 700–1,000 nm defocus yielding an effective pixel size of 2 Å. STEM: high angle annular dark field STEM images were captured on a JEM-2100F/Cs (JEOL) dedicated STEM with aberration correction. The probe size was set at 6c with a camera length of 12 cm and a beam current of 0.4 nA. Areas were scanned at X250,000 magnification and 4,096 × 4,096 pixels yielding a resolution of 2.2 angstroms per pixel. Both STEM and TEM images were analysed using ImageJ ( http://imagej.nih.gov/ij/ ) and lengths were recorded using the measuring tool. Total length was determined by tracing the proteins longest path. Hydrodynamic analysis S -value determinations were done using 5–20% sucrose density gradients in a volume of 12 ml. Protein samples at 0.1–0.3 mg were loaded into each tube. The standards used were all supplied from Sigma; cytochrome c, carbonic anhydrase, bovine serum albumin, β amylase, apoferritin, thyroglobulin. Centrifugation was carried out at 40,000 rpm at 4 °C for 20 h in a Beckman Ultracentrifuge in SW41Ti type rotor. Fractions of 250 μl were collected after the run. Each fraction was run on 10% SDS–PAGE and stained by Coomassie blue. The standard curves were drawn using the known S -values of the standard proteins and S -value of the unknown sample was calculated from this curve. For calculation of Stoke’s radius gel filtration chromatography was done using Superose6 GL10/30 column using protein standards. The molecular weight was then calculated using Siegel–Monty equation by using the Stoke’s radius and S -value found by these methods [9] . Native PAGE analysis Native PAGE was performed at eight different acrylamide concentrations for purified BASS (5 μg protein loaded into each lane) along with all the standards. Ferguson plots shows the relationship between relative mobility of BASS domain and acrylamide concentration and were drawn as semi logarithmic graph of 100 × log(100 × R f ) versus %T. The relationship between K r values determined for each standard protein and corresponding molecular weights were plotted in a logarithmic scale as a standard curve. Eight different standard proteins were analysed as was done for BASS. The standard proteins numbered as in Fig. 4c inset are (1) lactalbumin (14.2 kDa), (2) carbonic anhydrase (29 kDa), (3) chicken egg albumin (45 kDa), (4) BSA monomer, (5) BSA dimer, (6) catalase (250 kDa), (7) Urease trimer (272 kDa), (8) thyroglobulin dimer (330 kDa) and (9) thyroglobulin tetramer (660 kDa). The MW of BASS (and positive control fibrinogen) was calculated from this standard curve. Analytical ultracentrifugation All AUC measurements were performed in the UMC AUC facility in a Beckman Optima XLA analytical ultracentrifuge equipped with absorbance optics and an An60 Ti rotor. Sedimentation velocity data were collected at 50 K rpm, 20 °C at a wavelength of 280 nm using a spacing of 0.002 cm with one flash at each point in continuous scan mode. All sedimentation velocity data were initially analysed by DCDT + (version 1.15) to produce g(s) distribution plots. The weight average sedimentation coefficient values were obtained from DCDT + and corrected to S 20,w for the solution density and viscosity [44] . The density for each buffer was measured using an Anton Paar DMA 5000 density metre. CD spectral analysis All CD measurements were made on a Jasco J720 (We thank Wolfgang Kramer at Millsaps College for access to the CD instrument) at room temperature in a 0.2-mm path cell. Samples were diluted to appropriate concentrations and prespun in a TL 100 (TLA 100.2) at 100 K rpm for 5 min to remove aggregates, which otherwise cause significant variation in the signal intensity, especially at low I. Spectra on proteins and buffer were collected in triplicate from 260 to 190 nm for buffer correction. Mass spectral analysis Mass Spectrometric analyses of intact BASS were performed using a T-wave ion mobility mass spectrometry system, SYNAPT G2 HDMS (Waters Corp., Milford, MA) equipped with a nano-electrospray source. Under denaturing conditions, the protein was desalted using C4 Ziptip (EMD Millipore, Billerica, MA) and eluted into 50% acetonitrile/50% water/0.1% formic acid. Under native-like conditions, the protein was buffer-exchanged into 200 mM ammonium acetate (pH 6.8) using micro Bio-Spin P-6 columns (Bio-Rad, Hercules, CA) before mass spectrometric analysis. For each analysis, a 3–6 μl aliquot of the protein solution was loaded onto custom-made borosilicate glass nanotips. The acquisition parameters were adjusted to maintain the native state of ions without compromising the transmission efficiency and mass accuracy. Mass spectra were processed by MassLynx V4.1 (Waters Corp., Milford, MA). Site-directed spin labelling of BASS domain of kinesin-5 and EPR analysis The samples that were prepared for EPR analysis did not contain any DTT or β-mercaptoethanol in any of the buffer used. Instead tris(2-carboxyethyl)phosphine was used at a final concentration of 100 μM. The samples at protein concentrations between 1–2 mg ml −1 were labelled with MTSL (dissolved in acetonitrile and added to a final concentration of 300 μM). The excess spin label was removed by using Bio-Spin 6 Tris columns from Bio-Rad. An aliquot of purified, spin-labelled protein (5 μl) at a final concentration of ~100 μM protein was placed in a sealed quartz capillary contained in the resonator. Spectra of samples at room temperature (20–22 °C) were obtained by a single 60-s scan over 100 G at a microwave power of 2 milliwatts and a modulation amplitude optimized to the natural line width of 1 G. The protein concentration was determined by Bradford’s assay again for the analysed sample and this value was used for normalization of the EPR data. Rosetta modelling of kinesin-5 Homology and full atom modelling of Kinesin-5 was performed using the Rosetta homology [45] , [46] methods and X-ray structure of porcine cardiac tropomyosin (pdb id: 1C1G) [47] was used as a template. Chains A and B of BASS (residues 633–913 of full-length Kinesin-5) were modelled based on chains A and B (residues 2–282) of porcine cardiac tropomyosin, respectively. Ten thousand models of A and B chain complex were generated followed by model clustering as described previously [48] . The centre of the largest cluster model was selected as the best model. Dimer of dimers model was constructed manually using UCSF Chimera program [49] based on the EPR data suggesting proximity between residues 671 and 791 between dimers. How to cite this article: Acar, S. et al . The bipolar assembly domain of the mitotic motor kinesin-5. Nat. Commun. 4:1343 doi: 10.1038/ncomms2348 (2013).